Determination of collagen fibril size via absolute measurements of second-harmonic generation signals The quantification of collagen fibril size is a major issue for the investigation of pathological disorders associated with structural defects of the extracellular matrix. Second-harmonic generation microscopy is a powerful technique to characterize the macromolecular organization of collagen in unstained biological tissues. Nevertheless, due to the complex coherent building of this nonlinear optical signal, it has never been used to measure fibril diameter so far. Here we report absolute measurements of second-harmonic signals from isolated fibrils down to 30 nm diameter, via implementation of correlative second-harmonic-electron microscopy. Moreover, using analytical and numerical calculations, we demonstrate that the high sensitivity of this technique originates from the parallel alignment of collagen triple helices within fibrils and the subsequent constructive interferences of second-harmonic radiations. Finally, we use these absolute measurements as a calibration for ex vivo quantification of fibril diameter in the Descemet’s membrane of a diabetic rat cornea. Many pathological processes during development, wound healing or cancer are associated with the occurence of structural defects in collagen organization [1] , [2] . These defects are strikingly evidenced at the scale of fibrils that result from the alignment of collagen triple helices, with diameters of 10–300 nm, and dominate the structure of the extracellular matrix [3] , [4] . Quantification of collagen fibril size, density and organization is therefore a major biomedical issue. Since the demonstration of endogenous second-harmonic generation (SHG) from collagen fibrils [5] and the advent of multiphoton microscopy [6] , SHG microscopy has emerged as a powerful tool to visualize unstained fibrillar collagens within intact tissues [7] , [8] , [9] , [10] . Nevertheless, as an optical technique with typically 300 nm lateral resolution, SHG microscopy cannot resolve most of the collagen fibrils. Moreover, in contrast to incoherent fluorescence signals that scales linearly with the chromophore concentration, SHG is a coherent multiphoton signal that scales quadratically with the density of collagen triple helices aligned in a parallel way in the focal volume. Consequently, quantitative SHG measurements are highly challenging. From a physical point of view, SHG is usually associated to delocalized electrons in a noncentrosymmetrical environment giving rise to a first hyperpolarizability β at molecular scale. In biological tissues, the major molecular moieties exhibiting nonvanishing β are the peptide bonds along the protein backbones [11] , [12] , [13] , [14] . The SHG signal of collagen macromolecular assemblies is then obtained as the coherent summation of these elementary contributions. We have recently shown using hyper-Rayleigh scattering (HRS) experiments that the triple helix hyperpolarizability is built in a quantitative way from all its peptide bonds, as they are all aligned in the same direction without significant nonlinear interactions, and we have measured the first hyperpolarizability at the peptidic and molecular scales [14] . Nevertheless, applying such a quantitative bottom-up approach at the fibrillar scale raises the issues of the relative orientation and the interactions of collagen triple helices within a fibril. Moreover, its experimental validation requires the determination of the fibril diameter that is below the optical resolution, precluding quantitative SHG microscopy at the fibrillar scale so far. This paper presents the first absolute measurement of the SHG response of collagen fibrils and its dependence on fibril diameter. To that end, we implement correlative SHG-transmission electron microscopy (TEM) imaging by identifying sample preparation and excitation compatible with both techniques. We show that the SHG signal varies as the fourth power of the fibril diameter when smaller than the focal volume, validating the bottom-up approach at the fibrillar scale. In addition, this work determines the sensitivity threshold of SHG microscopy, that is the minimum size of fibril that can be detected using this technique. Finally, we show that these absolute measurements can be used as a reliable calibration for quantification of fibril diameter in an ex vivo biological tissue. Theoretical background Let us first derive an analytical expression of the SHG signal expected for a collagen fibril with diameter d in the focal plane of a nonlinear optical microscope (see Fig. 1 ). To that end, we use the paraxial approximation and consider forward SHG radiation excited by gaussian beams as Boyd et al. [15] The excitation beam propagates in the z direction and is focused within the two-dimensional collagen sample with lateral radius w 1 . The fibril is aligned along the x axis and exhibits a nonlinear optical susceptibility χ (2) characterized by a cylindrical symmetry around the x axis, with only two independent tensorial components: and . The laser is circularly polarized, which results in an effective susceptibility . We consider a pulsed laser with pulse duration τ , repetition rate R and mean power at focus P 1 . 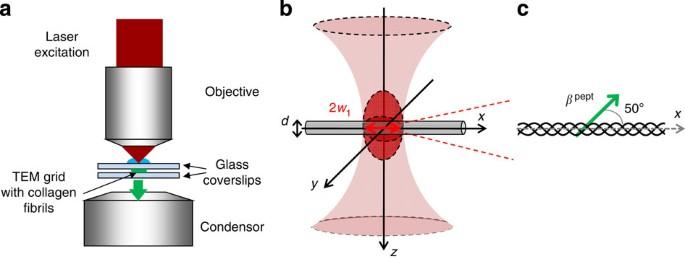Figure 1: Experimental setup and geometry. (a) SHG setup, (b) Collagen fibril in the focal volume, (c) Orientation of the microscopic hyperpolarizability. We then get the total number of SHG photons N SHG by integrating over the surface of the SHG beam at focus: Figure 1: Experimental setup and geometry. ( a ) SHG setup, ( b ) Collagen fibril in the focal volume, ( c ) Orientation of the microscopic hyperpolarizability. Full size image where indexes 1 and 2 correspond to fundamental and harmonic frequencies, respectively. λ stands for the wavelength, n for the refractive index. Δ t is the signal integration time, so that Rτ 1 Δ t corresponds to the actual illumination time. Finally, the last term takes into account the propagation of Gaussian beams: where Δ k is the phase matching parameter due to index dispersion and b is the confocal parameter (that is, depth of focus) of the incident Gaussian beam. The SHG signal depends on the fibril diameter d through the term in equation (1). As a working hypothesis, we suppose that the bottom-up approach applies at the fibrillar scale, which means that the fibril SHG response is obtained as the summation of the responses of all the triple helices that are considered as aligned in the same direction within the fibril with independent hyperpolarizabilities. Within this hypothesis, the fibril susceptibility is obtained as the product of the triple helix hyperpolarisability β mol (molecular scale) and the triple helices density in the fibril c mol . Note that this expression complies with the definition of a susceptibility that scales with the harmonophore density and does not depend on the sample dimension. Nevertheless, the diameter dependence lies in the heterogeneous response through the focal volume that may be larger than the fibril diameter. We then obtain a susceptibility equal to β mol c mol within the fibril and vanishing elsewhere, while equation (1) applies to a homogeneous effective susceptibility. To take into account this heterogeneity, we scale the fibril susceptibility by the ratio of the mean area section of the fibril to the one of the focal volume (with , the average thickness of the fibril along the optical axis z ). This phenomenological approach only applies for a fibril smaller than the waist diameter: d ≤2 w 1 , which ensures that S fib / S foc <1. One then gets: To highlight the diameter dependence of N SHG , we further simplify equation (1) by approximating the excitation field within the fibril as a plane wave for fibrils much smaller than the focal volume. It leads to and the more tractable equation: which reduces to: As expected, the SHG signal scales with the fourth power of the fibril diameter within this plane wave approximation. In practice, the full expression for gaussian beams (equation 1) provides a similar result for fibrils with diameter smaller than typically 250 nm as displayed in Fig. 2a . For larger fibrils, the gaussian calculation gives smaller SHG signals than the plane wave calculation. This is attributed to Gouy phase shift along the focus, which results in phase retardation of SHG waves radiated from either side of the focal plane and partly impedes coherent amplification of the SHG wave. Similar effects have been observed in corneas at the interface between two collagen lamellae [16] . 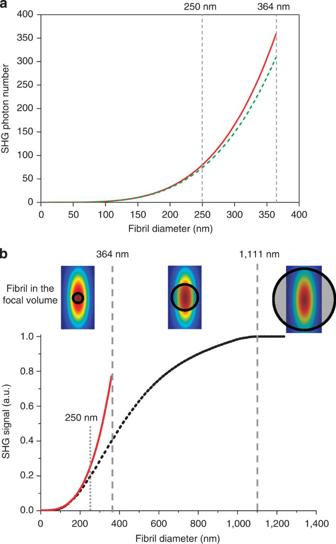Figure 2: Theoretical calculation of SHG signal as a function of the collagen fibril diameter. (a) Analytical calculation using plane wave approximation (red, straight line) or gaussian formalism (green, dotted line). (b) Numerical calculation (black dotted line) withd4fitting (red, straight line), for three diameter domains defined by the focal volume lateral and axial sizes (top). a.u., arbitrary unit. Figure 2: Theoretical calculation of SHG signal as a function of the collagen fibril diameter. ( a ) Analytical calculation using plane wave approximation (red, straight line) or gaussian formalism (green, dotted line). ( b ) Numerical calculation (black dotted line) with d 4 fitting (red, straight line), for three diameter domains defined by the focal volume lateral and axial sizes (top). a.u., arbitrary unit. Full size image Numerical calculation of fibril SHG signal Nevertheless, both the gaussian and simplified analytical expressions of the SHG signal exhibit several limitations. First, the way the fibril susceptibility is scaled by S fib / S foc to take into account the sample heterogeneity is a crude approximation, while effective to obtain analytical results. Second, these analytical expressions are derived in the paraxial approximation, although highly focused beam used for SHG imaging (numerical aperture (NA) ≈1.0) display a more complex intensity and phase distribution with various polarization components [17] . To overcome these limitations, we performed numerical simulations on the basis of a vectorial description of the electric fields and taking into account the spatial heterogeneity of the nonlinear response. The electric field distribution near the beam focus is calculated using the angular spectrum method [18] and the SHG signal distribution is obtained using all the components of the susceptibility tensor as detailed in ref. 17 . Notably, this approach accounts for polarization mixing due to strong focusing, including axial field components near the focus, and to phase variations within the focal volume. The nonlinear susceptibility is nonzero inside the fibril and vanishes elsewhere. The ratio of the two independent tensorial components is set to , in agreement with data obtained from polarization-resolved SHG microscopy [19] . Interestingly, this numerical calculation does not require S fib ≤ S foc and allows us to investigate the effect of the focal volume edges. Figure 2b displays the results of these calculations using Matlab software. The two vertical lines correspond to the lateral (364 nm) and the axial (1,111 nm) diameter (at 1/e) of the focal volume, considering 860-nm excitation focused by × 40, 1.1 NA water-immersion objective and neglecting any aberration. For small fibril diameters ( d <250 nm), the SHG signal varies approximately as d 4 in good agreement with the analytical calculation. For intermediate fibril size (250 nm< d <1,111 nm), the SHG signal increasing rate is much smaller than d 4 . Indeed, the collagen molecules responsible for the diameter increase contribute moderately to the SHG signal because they lie at the edges of the focal volume where the excitation power is smaller and eventually vanishes. Finally, the SHG signal reaches a plateau when the fibril is larger than the focal volume. Importantly, for fibril diameters <250 nm, that is most of the collagen fibrils (diameter 10–300 nm), these numerical simulations confirms the d 4 dependence of the SHG signal obtained by the analytical approach. Correlative SHG-electron microscopy To validate these analytical and numerical calculations, we implemented correlative SHG-electron imaging on isolated collagen fibrils. To that end, we used fibrils synthetized in vitro from acidic collagen extracted from rat-tail tendons, which exhibit exactly the same periodic structure as native collagen fibrils [3] and are widely used as biomimetic matrices. A low-density solution of fibrils with tailored diameters was thus obtained upon pH increase in controlled conditions (see Methods) [20] , [21] . Fibrils were deposited on a numbered TEM finder grid and dried in air. The grid was first visualized by SHG microscopy, and then by TEM, without any further staining or fixation step. We found that moderate laser excitation power (typically 12 mW) combined with the use of carbon-free gold grids was mandatory for limiting laser damage due to excessive heating of the TEM subtrates during SHG imaging. 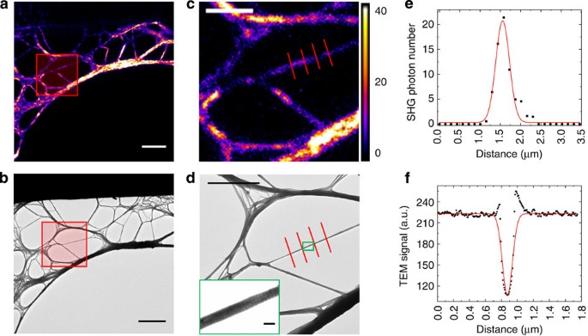Figure 3: Correlative SHG-electron imaging. (a) SHG and (b) TEM images of unstained collagen fibrils (scale bar, 10 μm). (c,d) Zoomed regions of interest from (c) SHG and (d) TEM images (scale bar, 5 μm). The inset in the TEM image shows a striated fibril (scale bar, 0.2 μm). (e) Intensity profile of SHG signal along one red line inc(black square) with gaussian fitting (red curve). (f) Same for TEM signal along one red line ind. Note that the upper values at the fibril edges in the TEM profile are due to slight defocusing of the electron beam to enhance contrast. a.u., arbitrary unit. Figure 3a–d present typical correlative images. The TEM image displays the same distribution of fibrils as the SHG image, which shows that the vacuum drying step does not modify the sample structure significantly. The very same fibrils can be observed with the two imaging techniques with the help of the grid markers (see Fig. 3a–d ). Figure 3: Correlative SHG-electron imaging. ( a ) SHG and ( b ) TEM images of unstained collagen fibrils (scale bar, 10 μm). ( c , d ) Zoomed regions of interest from ( c ) SHG and ( d ) TEM images (scale bar, 5 μm). The inset in the TEM image shows a striated fibril (scale bar, 0.2 μm). ( e ) Intensity profile of SHG signal along one red line in c (black square) with gaussian fitting (red curve). ( f ) Same for TEM signal along one red line in d . Note that the upper values at the fibril edges in the TEM profile are due to slight defocusing of the electron beam to enhance contrast. a.u., arbitrary unit. Full size image The fibril diameter is then measured on the TEM images. Transverse profiles at four different positions are fitted by gaussian functions to calculate the mean diameter and standard deviation over the fibril length. The SHG signal is measured the same way at the same four positions approximately ( Fig. 3e,f ). The width of the SHG profile gives the optical resolution, but the gaussian maximum intensity provides the SHG photon counts for this fibril. Such measurements were performed in six different samples for a total of 146 fibrils. Fig. 4a displays the SHG photon counts as a function of the fibril diameters for one grid. It shows that we successfully obtained fibrils with various diameters in the 30–250 nm range, and provides two types of information. First, we can estimate the sensitivity of SHG microscopy. In our setup, the smallest observable fibril has a diameter of 30 nm. Smaller fibrils were imaged by electron microscopy, but did not exhibit SHG signals above the noise level. Note that the main limitation is the photodamage of the fibrils due to residual absorption, which constrains the excitation power and integration time. Nonetheless, SHG microscopy appears as a highly sensitive technique that can detect almost all fibrils in tissues. This sensitivity threshold of 30 nm can be translated to the molecular scale considering the molecular density of collagen fibrils ( c mol =1.3 × 10 24 m −3 ; ref. 4 ), which gives a minimum of 390 triple helices. Considering the [( Gly − X − Y ) 337 ] 3 structure of type I collagen, we further find that a minimum of 1.2 × 10 6 peptide bonds is required to generate detectable SHG signals. 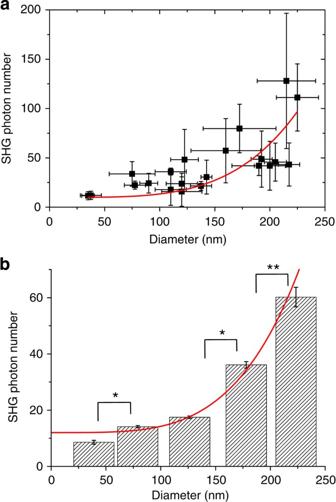Figure 4: Calibration of collagen SHG signal. SHG photon number as a function of the fibril diameter measured on the TEM image for (a) one sample and (b) all samples using diameter bins of 50 nm. Red lines correspond to allometric fitting. The error bar is the standard deviation over four measures along four different profiles in the same fibril inaand the s.e.m. over all fibrils in the same bin inb(6 to 35 fibrils per bin). *P<0.05, **P<0.01 using sided two-sample Welsh’st-test. Figure 4: Calibration of collagen SHG signal. SHG photon number as a function of the fibril diameter measured on the TEM image for ( a ) one sample and ( b ) all samples using diameter bins of 50 nm. Red lines correspond to allometric fitting. The error bar is the standard deviation over four measures along four different profiles in the same fibril in a and the s.e.m. over all fibrils in the same bin in b (6 to 35 fibrils per bin). * P <0.05, ** P <0.01 using sided two-sample Welsh’s t -test. Full size image Second, our correlative data enable the calibration of SHG signal as a function of the fibril diameter. To that end, we merged the data of all six samples and gathered the 146 fibrils into 50-nm diameter bins (see Fig. 4b ). Fifty nanometres appeared as the minimal binning size to obtain statistically distinct SHG signals, with small s.e.m. This calibration curve then enables to retrieve the fibril diameter from the SHG signal with ±25 nm accuracy without any TEM imaging. Finally, to verify our theoretical analysis, we fitted the correlative data using an allometric function as in equation (5): N SHG = N 0 + B . d 4 where N 0 is the background noise. We obtained satisfactory coefficients of determination ( R 2 =0.91 for Fig. 4b ), showing that our measurements exhibit a d 4 dependence as expected from equation (4). Alternatively, we fitted the calibration data using a free exponent and obtained values close to 4 (3.83 for Fig. 4b ). Most importantly, the allometric parameter B provides a quantitative value of the effective hyperpolarizability at molecular scale . Using equation (5), we get: where A is the numerical parameter in equation (4) and η =18% is the detection efficiency of our setup. This parameter takes into account the losses in the detection path and the quantum yield (20%) of the photomultiplier tubes. A is calculated from equation (4) using fundamental constants and experimental parameters: repetition rate R =76 MHz , pulse duration τ 1 =150 fs , integration time Δ t =10 μs, laser wavelength λ 1 =860 nm, power at focus P 1 =12 mW, n 1 =1.47, n 2 =1.5 and focal volume 1/e half-width w 2 =220 nm. Importantly, A is inversely proportional to . Reliable calibration therefore requires an accurate measurement of this parameter that is highly sensitive to aberrations, mostly due to the thin air layer between the two glass coverslips. Table 1 displays the values of B and of obtained when fitting the data of every grid or all data together, either using diameter bins or not. We obtain reproducible data, leading to . Table 1 Absolute measurements of collagen hyperpolarizability. Full size table Quantification of fibril size in a biological tissue As a proof of feasibility, we applied this SHG signal calibration to determine the diameter of hyperglycemia-induced collagen fibrils observed in the Descemet’s membrane of an unfixed rat cornea. The Descemet’s membrane is located in the posterior part of the cornea, near the endothelium, and is mainly composed of non-fibrillar collagens that form centrosymmetrical networks and do not exhibit any SHG signal. However, sparse collagen fibrils were recently evidenced in the Descemet’s membrane of diabetic rat corneas, as well as other hyperglycemia-induced structural corneal abnormalities [22] , [23] , [24] . 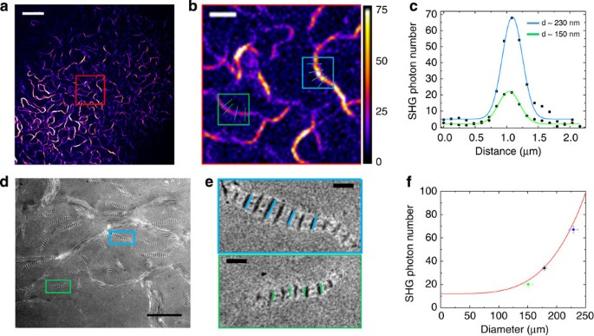Figure 5: Quantification of fibril diameter in an unfixed diabetic rat cornea. (a)Ex vivoSHG image of the Descemet’s membrane (scale bar, 50 μm) and (b) zoomed region of interest with fibrils exhibiting low (green) or high (blue) SHG signal (scale bar, 10 μm). (c) SHG intensity profiles in fibrils highlighted in blue and green colour inb, with gaussian fitting. (d) TEM image of an ultrathin frontal section of the same region of the same cornea (scale bar, 2 μm) and (e) zoomed images of typical small (green) and large (blue) collagen fibrils (scale bar, 0.2 μm). (f) SHG photon number derived fromcas a function of the fibril diameter measured ind, superimposed to the SHG calibration curve (red line). The black data point corresponds to SHG and TEM data measured in serial transverse sections of the same cornea. Error bars correspond to s.e.m. (five samples for small or large fibrils in intact cornea, three samples for serial transverse section). Figure 5a,b display ex vivo frontal SHG images of these fibrils in an intact cornea. To determine the fibril diameter, we measured the SHG photon numbers in the same way as for synthetized collagen fibrils (see Fig. 5c ). These results were then corrected for the different imaging conditions using equation (4): Figure 5: Quantification of fibril diameter in an unfixed diabetic rat cornea. ( a ) Ex vivo SHG image of the Descemet’s membrane (scale bar, 50 μm) and ( b ) zoomed region of interest with fibrils exhibiting low (green) or high (blue) SHG signal (scale bar, 10 μm). ( c ) SHG intensity profiles in fibrils highlighted in blue and green colour in b , with gaussian fitting. ( d ) TEM image of an ultrathin frontal section of the same region of the same cornea (scale bar, 2 μm) and ( e ) zoomed images of typical small (green) and large (blue) collagen fibrils (scale bar, 0.2 μm). ( f ) SHG photon number derived from c as a function of the fibril diameter measured in d , superimposed to the SHG calibration curve (red line). The black data point corresponds to SHG and TEM data measured in serial transverse sections of the same cornea. Error bars correspond to s.e.m. (five samples for small or large fibrils in intact cornea, three samples for serial transverse section). Full size image where ′ denotes the acquisition settings for ex vivo cornea imaging compared with the ones for synthetized fibrils: integration time Δ t ′=4 μs, laser wavelength , power at focus , and focal volume 1/e half-width w ′ 2 =200 nm. To validate these results, we measured the diameter of fibrils by the use of TEM in ultrathin frontal sections of the same region of the same cornea as depicted in Fig. 5d,e . Note that direct correlation to SHG image of the very same fibrils was not possible because of the specific cornea preparation for TEM (paraffin embedding, slicing). We then plotted the corrected SHG photon number as a function of the fibril diameter for two populations of fibrils, that is wide fibrils with high SHG signals and thin fibrils with low SHG signal (averaged value and s.e.m. over five different fibrils). Comparison with the calibration curve showed a good agreement as displayed in Fig. 5f . However, the measured SHG photon numbers were slightly smaller than the ones expected from the calibration curve, which may be attributed to a deterioration of the SHG collection when detecting through the entire rat cornea (thickness ≈200 μm ) compared with thin samples. To address this question, we acquired SHG images in a thin transverse section of the diabetic cornea and compared it with TEM images of a serial ultrathin section. Due to the small numbers of fibrils visualized in this geometry, we averaged measurements only on three typical fibrils using both techniques. After correction of the acquisition settings, it provided the data depicted in black in Fig. 5f , which exhibits an excellent agreement with the calibration. It demonstrates the validity of our calibration for samples with equivalent detection efficiency. In this paper, we reported absolute measurements of SHG signal from collagen fibrils of tailored diameters by the use of correlative SHG-electron imaging. This correlative approach was mandatory to measure the SHG signal and the fibril diameter on the very same fibril. While correlative confocal-electron imaging has been reported [25] , only comparative SHG-electron imaging coupled with statistical analysis has been used so far. Alternatively, correlation of SHG microscopy to atomic force microscopy has been reported, but only for a few fibrils in a dense matrix, allowing no accurate calibration and no assessement of the sensitivity threshold [26] . In this study, we identified the appropriate conditions to achieve SHG microscopy on fibrils prepared for TEM, that is typically a few mW excitation power and carbon-free gold grids. Our correlative SHG-electron data allowed us to determine the sensitivity threshold of SHG microscopy in terms of fibril diameter: 30 nm, and of peptide bonds number: 1.2 × 10 6 in our setup. It proves that SHG microscopy is a sensitive imaging technique that can detect signals from collagen fibrils 15 times smaller than the optical resolution. Such a high sensitivity is quite unique considering that it applies to an endogenous signal, with no labelling of collagen fibrils. Most importantly, correlative imaging enabled the calibration of the SHG signal as a function of the fibril diameter with ±25 nm accuracy. Although it only applies to our specific experimental conditions, this calibration can be adapted in a straightforward way to fit any change of the acquisition parameters or imaging in another setup. For instance, variation of the excitation power or the detection integration time may be taken into account using equation (4). Alternatively, fixed reference samples may be used to calibrate other setups relative to ours. This calibration could also be generalized to three-dimensional samples in a straightforward way by imaging the out-of-plane angle of the fibril and including appropriate tensorial response in equation (1) [27] , [28] . The applicability of this calibration to SHG images of unfixed thick biological tissues was demonstrated in a diabetic rat cornea exhibiting sparse collagen fibrils in the Descemet’s membrane. This tissue was chosen because it advantageously exhibits no absorption or scattering, facilitating the application of the calibration. The diameter of the fibrils in the Descemet’s membrane was deduced from the signal intensity in the SHG image by use of the calibration and compared with TEM measurements in an ultrathin section of the same cornea. We obtained a good agreement, proving the reliability of the calibration in thick biological samples. Nevertheless, the fibril diameter was slightly underestimated due to lower SHG collection efficiency in intact cornea compared with a thin sample. In a more general way, propagation effects in biological tissues such as absorption, scattering and aberrations may significantly change the power at focus, the size of the focal volume and the signal collection, which is critical in the SHG signal calibration. Such effects could, however, be taken into account by Monte-Carlo simulations, while certainly limiting the accuracy of processed quantitative data [29] , [30] . From a fundamental perspective, we also deciphered the physical origin of the diameter dependence and the high sensitivity of SHG signals in fibrils by using a bottom-up approach of the fibril susceptibility and deriving an analytical expression of the SHG signal from collagen fibrils with various diameters. This expression provided a d 4 dependence, which was confirmed by numerical calculations taking into account, in a more rigourous way, strong focusing in a sub-micrometer-sized sample. Our experimental results were in good agreement with this theoretical analysis. The calibration data then provided a measurement of the collagen effective hyperpolarizability at a molecular scale in our experimental conditions, that is with circular excitation and trans-detection of SHG signal. This result must be compared with recent measurements of collagen hyperpolarizability using HRS [12] , [14] . As the effective molecular hyperpolarizability measured by HRS does not correspond to the same polarization and setup geometry as in SHG microscopy, we look at the peptide bond scale. Duboisset et al. [14] obtained β pept,HRS =(2.8±0.4) × 10 −40 m 4 V −1 by considering that the molecular hyperpolarizability tensor corresponds to the summation of peptide bond responses oriented at 50° angle to the triple helix axis (see Fig. 1c , 3,033 peptide bonds per collagen I triple helix). This effective pitch angle is obtained from polarization-resolved SHG measurements, in agreement with the theoretical calculations [13] , [19] . Applying the same approach to SHG geometry (see Fig. 1b , circular polarization), the peptide bond hyperpolarizability calculated from our data is β pept,SHG =(2.9±0.3) × 10 −40 m 4 V −1 , in excellent agreement with the HRS data. This result therefore validates our theoretical calculation building up the fibril susceptibility from the molecular response. It indicates that all the triple helices are aligned in the same direction within a fibril and do not interact in a significant way regarding their nonlinear optical response. Notably, antiparallel collagen molecules within the same fibril would have resulted in partly destructive interferences of their SHG radiation and consequently smaller apparent peptide hyperpolarizability. Importantly, this unipolar fibrillar organization deduced from our absolute measurements is consistent with ultrastructural studies at nanometre scale by the use of TEM [31] or atomic force microscopy [32] . Fibril polarity reversal has nevertheless been observed in fibrils extracted from some embryonic tissues, but it occurs in a small transition region (about 0.5 μm) along the fibril [31] , which should not impede quantitative SHG measurements along the main part of the fibril. Altogether, our data show that the high sensitivity of SHG microscopy to collagen fibrils is inherently related to the parallel alignment of collagen molecules within the same fibril that ensures fully constructive interferences of the SHG radiations from all the peptide bonds within the fibril. Note that the same mechanism does not apply to the fibre or fascicle scale because the fibrils may be oriented in antiparallel directions within a fibre or any dense collagen tissue. Such an antiparallel organization was recently demonstrated in a direct way by the use of piezoelectric microscopy [33] . It results in partially destructive interferences in the forward direction and decreases the forward-detected SHG signal compared with the signal expected for parallel fibrils [5] , [27] , [33] , [34] , [35] . The forward-detected SHG signal is then still larger than the backward-detected one, but the ratio of these signals is not as high as expected from the ratio of the coherence lengths in forward and backward directions, in agreement to measures in tissues such as tendons or fascia [35] , [36] , [37] . Quantitative SHG data at the tissular scale are therefore highly sensitive to the collagen density and organization in the focal volume [8] , [27] , [29] , [33] , [34] , [35] , [38] . In other words, our calibration is not based on a super-resolution technique and only applies to low-density matrices or tissues where the distance between two fibrils is larger than the optical resolution, so that there is only one fibril in the focal volume, with all the collagen molecules pointing in the same direction. Nevertheless, complementary approaches may be used to quantify dense collagen distributions in tissues, by combining numerical calculation and measurements sensitive to the collagen organization within the focal volume as recently reported [35] . Indeed, given a specific distribution of collagen fibrils within the focal volume (filling fraction, diameter and direction of fibrils), the overall SHG signal can be calculated as the coherent summation of the SHG response of each fibril and compared with polarization-resolved measurements, interferometric measurements or comparative forward/backward detection that provide additional information about collagen distribution at sub-micrometer scale [19] , [29] , [35] , [39] , [40] . Altogether, we are quite confident that quantitative SHG imaging will be ultimately achieved in most collagen-rich biological tissue on the basis of our calibration on isolated fibrils. In conclusion, this paper reports the calibration of collagen SHG signal at fibrillar scale by the use of correlative SHG-electron imaging. We showed that SHG signals vary as the fourth power of the fibril diameter and that the sensitivity threshold is as low as 30 nm because all the triple helices are aligned in the same direction within a fibril, so that their contributions interfere constructively. This calibration was subsequently used to determine the size of hyperglycemia-induced collagen fibrils in the Descemet’s membrane of a rat cornea. Altogether, those results represent a major step for advanced biomedical studies that require in situ quantification of collagen fibrils in intact tissues. Such a quantitative SHG microscopy should serve as a sensitive diagnosis of collagen remodelling in many pathologies. Collagen sample preparation Type I collagen was extracted and purified from rat-tail tendons [41] . Briefly, fresh tendons were washed with phosphate-buffered saline solution and solubilized in 0.5 M acetic acid. The crude solution was centrifuged and the supernatant was selectively precipitated with 0.7 M NaCl. Precipitated type I collagen was solubilized in 0.5 M acetic acid, then desalted by dialysis against 0.5 M acetic acid. Sample purity was assessed by electrophoresis and the concentration estimated by hydroxyproline titration. All other chemicals were purchased and used as received. Water was purified with a Direct-Q system (Millipore Co.). Collagen (100 μg ml −1 ) was then solubilized in 0.5 M acetic acid (pH=2.5, final volume V f =100 μl) and fibrillogenesis was triggered upon increasing pH by ammonia diffusion for 1 h (ref. 21 ). A small drop of sample (3 μl) was placed on a numbered TEM gold finder grid (200 mesh) without carbon coating and dried in air during one day. The grid was then clamped between two glass coverslips (about 5 μm spacing) and the sample was directly visualized using SHG microscopy without any staining. SHG microscopy Multiphoton imaging was performed using a custom-built laser scanning microscope [9] , [16] , based on a femtosecond Ti-Sapphire laser (Tsunami, Spectra-Physics). Samples were illuminated in an upright geometry using quasi-circularly polarized excitation at 860 nm (ellipticity 0.88) to enable homogenous imaging of fibrils whatever their orientation in the focal plane. SHG signals were recorded in the forward direction using photon-counting photomultiplier tubes (P25PC, Electron Tubes) with appropriate spectral filters (FF01-680/SP, FF01-720/SP and FF01-427/10, Semrock). High NA water-immersion objective ( × 40, NA 1.10, LD C-Apochromat, Zeiss) was used to focus the laser beam, with typically 12 mW laser power at the objective focus. As the ≈5 μm-thick air layer between the two coverslips introduced aberrations, we directly measured the focal volume radius on intensity profiles of the smallest fibrils and obtained w 2 =220 nm (diameter at 1/e: 440 nm). SHG image stacks were recorded at 100 kHz pixel rate every 0.5 μm in the axial direction, using 0.175 μm lateral pixel size, to be sure to capture the signal maximum. SHG image of a fibril was then obtained as the maximum intensity projection of the z-stack and used without any filtering. Transmission electron microscopy Whereafter, the same grid was imaged using a JEOL 1011 electron microscope operating at 100 kV and equipped with a Gatan Orius CCD camera. Identifying the markers on the grid ensured to image the same fibrils as with SHG microscopy. Importantly, the only operation between SHG and TEM imaging was placing the sample under vacuum in the electron microscope at room temperature, without any staining or fixation steps. As collagen sample was dried before SHG imaging, SHG and TEM images are acquired on fibrils with the same hydration state and consequently the same diameter, considering that the vacuum step does not modify the fibril size in dehydrated samples. SHG imaging of rat cornea Corneas from a 1-year-old Goto-Kakizaki rat, a spontaneous model of type 2 diabetes, were studied in the framework of a project about hyperglycemia-induced corneal abnormalities [23] , [24] . This study was performed in accordance with the ARVO Statement for the Use of Animals in Ophthalmic and Research Vision. The corneas were removed just after the killing of the rat and they were mounted between two glass coverslips with a drop of Hanks medium for ex vivo frontal imaging (no fixation). Multiphoton image stacks were acquired on the full depth of the cornea (endothelium up) using the same setup as for collagen fibrils (see above). The excitation wavelength was set to 730 nm to enable imaging of cellular endogenous fluorescence when necessary, with 30 mW excitation power at the objective focus. We used a × 60, NA 1.2 water-immersion objective (Olympus), with 2 w ′ 2 ≈400 nm. SHG was detected in the forward direction with suitable spectral filters (FF01-680/SP, FF01-720/SP and Hg01-365-25, Semrock). Images were acquired at 250 kHz pixel rate, every 0.5 μm in the axial direction and using 0.130 μm lateral pixel size. Other acquisition settings were similar to the ones specified for isolated collagen fibrils. After multiphoton imaging, the cornea was fixed and oriented regions of interest were included in epoxy resin as reported in ref. 24 . Ultrathin frontal sections were stained with uranyl acetate and lead citrate and observed with TEM (TEM CM10, Philips). Alternatively, ultrathin transverse sections were stained the same way for TEM imaging and compared with SHG imaging of serial thin sections [23] . How to cite this article: Bancelin, S. et al. Determination of collagen fibril size via absolute measurements of second-harmonic generation signals. Nat. Commun. 5:4920 doi: 10.1038/ncomms5920 (2014).